Evidence for interacting two-level systems from the 1/fnoise of a superconducting resonator The performance of a great variety of electronic devices—ranging from semiconductor transistors to superconducting qubits—is hampered by low-frequency noise with spectra proportional to 1/ f . The ubiquity and negative impact of 1/ f noise has motivated intensive research into its cause, and it is now believed to originate from a bath of fluctuating two-level defect states (TLSs) embedded in the material. This phenomenon is commonly described by the long-established standard tunnelling model (STM) of independent TLS. A key prediction of STM is that the noise should vanish at low temperatures. Here we report measurements on superconducting microresonators over previously unattainable, very long time scales that show an increase in 1/ f noise at low temperatures and low microwave power, contrary to the STM. We propose a new generalised tunnelling model that includes significant interaction between multiple TLSs, which fully describes these observations, as well as recent studies of individual TLS lifetimes in superconducting qubits. Initially introduced to explain unusual thermal properties of glasses with respect to crystals, the standard tunnelling model (STM) [1] , [2] has enjoyed considerable success in describing many other phenomena in both ordered and disordered systems. The STM assumes the ability for a number of atoms at low temperatures to quantum mechanically tunnel between adjacent lattice sites. The model has since then been adopted to describe two-level defect states (TLSs) in many other contexts: for example, TLS can be caused by tunnelling of electrons in insulating barriers, molecules with two quasi-stable configurations and so on [3] , [4] , [5] . More generally, any influence of dilute impurities on macroscopic properties of materials is often parametrized as a bath of non-interacting TLSs, such that the STM is applicable. In particular, TLSs have been suggested as sources of the ubiquitous 1/ f noise in electronic materials [6] and are also active at low temperatures, where the kinetics is dominated by tunnelling [7] , [8] . With the rapid recent progress of new devices for quantum information processing and detector applications, there is a renewed awareness [9] of the deleterious effects of TLS noise. Here we demonstrate theoretically and experimentally that the STM fails in the extreme low temperature, low-power limits where these new devices are typically operated; therefore, an extension of STM to include specific interactions between TLSs is necessary to address the shortcomings of this tried and trusted model. The properties of TLSs can be conveniently studied using thin-film high-quality superconducting microwave resonators, which by themselves are important for a number of diverse applications ranging from quantum computation [10] to submillimetre and far-infrared astronomy [11] . Here TLSs, mainly located at interfaces, cause 1/ f noise that manifests as an instability in the centre frequency. The mechanism can be understood by noting that TLSs behave as an ensemble of switching dipoles resulting in a fluctuating dielectric constant and induced electric noise in the resonator. Device performance can be severely hampered by the resulting jitter. Since a study of low-frequency noise requires measurements that span a long time, the effects due to TLSs are often masked by unrelated instabilities in the resonator and the measurement system. There have been a number of studies of TLS noise in superconducting resonators [12] , [13] , [14] , [15] , [16] , [17] to date; however, these results have not been explainable within the STM. This has motivated the development of new models that either assume the presence of additional sources of dissipation , for example, caused by edge defects [18] or, alternatively, explain the shortcomings of the STM by re-evaluating the underlying assumptions about the nature of TLS. Here we demonstrate that the noise of superconducting microresonators [19] increases as the temperature is decreased, an observation in direct contradiction to the STM. To account for these results we propose a new model, which includes significant interactions between TLSs. The interactions lead to spectral diffusion that alters the properties of the resonator. We show that besides explaining our results, the new model also explains results of other recent studies [20] that used phase qubits as a way to probe individual TLS. We emphasize that these measurements were made possible through the use of an ultrastable Pound loop frequency-tracking technique [21] and specially designed low-noise epitaxial superconducting resonators with high temperature stability. Experimental results We have performed a detailed study and analysis of the very low-frequency noise in high-quality Nb resonators. These measurements were performed in various microwave powers, down to average energies corresponding to ‹ n ›=1−10 photons in the resonator. A crucial feature of our measurements is the long measurement time ( τ >10 4 s) leading to high statistical confidence. Two devices with different resonance frequencies, denoted Res1 and Res2, are studied in detail. The resonators (shown in Fig. 1a ) are made of 50-nm-thick epitaxial Nb film with a 5-nm Pt-capping layer grown by laser ablation on r-plane sapphire (see Methods for details). The resonators have centre frequencies ( ν 0 ) between 4–8 GHz, and intrinsic quality factors ( Q ) above 10 5 . 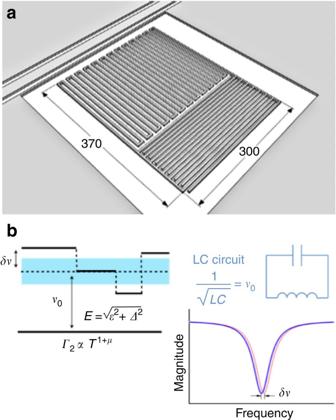Figure 1: Experimental overview. (a) Layout of a superconducting resonator comprising an interdigital capacitor and an inductive meander. The metallization layer is shown in grey and exposed substrate is shown in white. All dimensions are in micrometre and the lines are 4-μm wide. The resonator is inductively coupled to a coplanar feedline. (b) Conceptual model for the noise: quantum coherent TLS with energy splittingE≈ν0acquires a widthΓ2∝T1+μbecause of dipole–dipole interactions with a bath of TLSs having density of statesρ(E)∝Eμ. Hereμ≈0.3 andTis temperature. The resonant coherent TLSs are in turn affected by surrounding classical fluctuators strongly coupled to them that cause an energy drift, bringing the resonant TLS in and out of resonance. The LC resonator is sensitive to this energy drift and the result is a frequency shiftδν, shown in the magnitude response. Further parameters can be found in Table 1 in the Methods section. Figure 1: Experimental overview. ( a ) Layout of a superconducting resonator comprising an interdigital capacitor and an inductive meander. The metallization layer is shown in grey and exposed substrate is shown in white. All dimensions are in micrometre and the lines are 4-μm wide. The resonator is inductively coupled to a coplanar feedline. ( b ) Conceptual model for the noise: quantum coherent TLS with energy splitting E ≈ ν 0 acquires a width Γ 2 ∝ T 1+ μ because of dipole–dipole interactions with a bath of TLSs having density of states ρ ( E ) ∝ E μ . Here μ ≈0.3 and T is temperature. The resonant coherent TLSs are in turn affected by surrounding classical fluctuators strongly coupled to them that cause an energy drift, bringing the resonant TLS in and out of resonance. The LC resonator is sensitive to this energy drift and the result is a frequency shift δν , shown in the magnitude response. Full size image Table 1 Device parameters for the resonators used in this work. Full size table The measurements were performed by continuously monitoring the time-varying centre frequency ν 0 ( t ). For all measurements presented in this work, the quantity of interest is the fractional frequency spectra ( S y in units of 1/Hz), which is defined by , where S d ν is the frequency spectra (in units of Hz 2 /Hz), ν 0 is the nominal centre frequency of the resonator and f ( t i ) the Fourier frequency (see Methods for details). The central result of this work is presented in Fig. 2 , which shows the level of 1/ f noise at 0.1 Hz plotted for the temperature range 60–500 mK at three different microwave drive levels; examples of full spectra can be found in Fig. 3a . For both resonators we find a stronger than 1/ T temperature dependence for all microwave drives. These data can be fit to S y ( T ) ∝ a / T 1+ μ , where a is a power-dependent constant and μ =0.22±0.16 and μ =0.36±0.3 for Res1 and Res2, respectively. Hence, both sets of measurements suggest a temperature dependence stronger than 1/ T . As will be shown later, μ turns out to be a microscopic parameter that can be directly related to the density of states of TLSs. 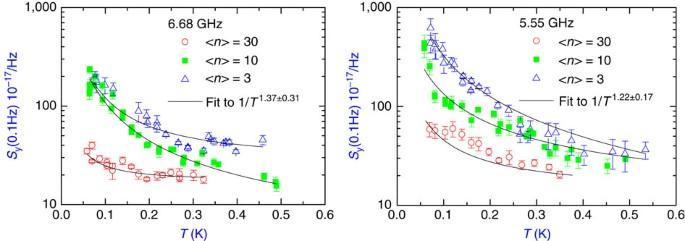Figure 2: Temperature dependence of 1/fnoise in superconducting microresonators. The 1/fnoise is measured atSy(0.1 Hz) in varying temperature and for different average photon energies in the resonator. The solid line is a fit to a power law highlighting an inverse temperature dependence. The noise saturates at a power-dependent level above the system noise floor ofSy(0.1 Hz)=5 × 10−17. The error bars indicate type A uncertainties from the propagated error of the fitting process. Figure 2: Temperature dependence of 1/ f noise in superconducting microresonators. The 1/ f noise is measured at S y (0.1 Hz) in varying temperature and for different average photon energies in the resonator. The solid line is a fit to a power law highlighting an inverse temperature dependence. The noise saturates at a power-dependent level above the system noise floor of S y (0.1 Hz)=5 × 10 −17 . The error bars indicate type A uncertainties from the propagated error of the fitting process. 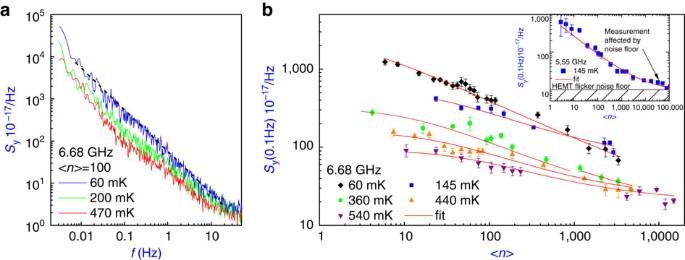Figure 3: Microwave drive and temperature dependence of 1/fnoise in superconducting microresonators. (a) Fractional frequency spectra at three different temperatures for resonator Res2. For frequencies below 10 Hz the slope is −0.97 with a goodness-of-fit parameterR2=0.9, white noise dominates from 50 Hz. (b) 1/fnoise level versus average number of photons within the resonator Res2 at several different temperatures. The average photon number is calculated as ‹n›=Wsto/ħ, whereħis Planck’s constant,ω0is the resonators centre frequency and, wherePappis the applied microwave drive andSmin21is the magnitude of the resonance dip. The data are fit to the noise spectra calculated from the model. Inset: 1/fnoise versus average number of photons for resonator Res1 showing the leveling off at high photon numbers (high microwave drive) that is because of flicker noise floor of the amplifier chain. The error bars indicate type A uncertainties from the propagated error of the fitting process. Full size image Figure 3: Microwave drive and temperature dependence of 1/ f noise in superconducting microresonators. ( a ) Fractional frequency spectra at three different temperatures for resonator Res2. For frequencies below 10 Hz the slope is −0.97 with a goodness-of-fit parameter R 2 =0.9, white noise dominates from 50 Hz. ( b ) 1/ f noise level versus average number of photons within the resonator Res2 at several different temperatures. The average photon number is calculated as ‹ n ›= W sto / ħ , where ħ is Planck’s constant, ω 0 is the resonators centre frequency and , where P app is the applied microwave drive and S min 21 is the magnitude of the resonance dip. The data are fit to the noise spectra calculated from the model. Inset: 1/ f noise versus average number of photons for resonator Res1 showing the leveling off at high photon numbers (high microwave drive) that is because of flicker noise floor of the amplifier chain. The error bars indicate type A uncertainties from the propagated error of the fitting process. Full size image We also find that the 1/ f noise level depends on the microwave drive or, more precisely, on the energy stored in the resonator, consistent with our previous results [17] . At the highest powers (inset of Fig. 3b ), we also see a saturation due to amplifier noise at a level consistent with other estimates [18] , [22] . However, Fig. 3 shows that as power is decreased the resonator noise increases, until it saturates in the low power limit, at a level found to be temperature-dependent. Examining possible noise mechanisms We first discuss whether the jitter in the resonator frequency could be caused by inductance fluctuations from surface spins. The argument in favour of this is that inductance fluctuations according to ref. 23 exhibit a 1/ f frequency dependence for T ≲ 200 mK and that the noise level increases as the temperature is reduced in the range 100< T <2 K. However, it is to be noted that the details of the behaviour are very different to our observations: inductance noise acquires an approximate 1/ f dependence only at the lowest temperatures, while at higher temperatures it is described by a much smaller exponent [24] . Furthermore, at f ~1 Hz the inductance noise is almost temperature-independent and, crucially, for all frequencies the temperature dependence ceases below T ≲ 200 mK. Finally, the power saturation of the noise seen in our resonators ( Fig. 3b ) implies that the frequency of the relevant excitation is close to the frequency of the resonator—for example, f ~6 GHz. These frequencies are too large for a dilute spin system with the densities consistent with direct observations [23] , [24] . To completely rule out spin as the dominant source of jitter, we performed measurements in weak (≈mT) in-plane fields, which would be expected to affect these spin systems, but not the superconductor [25] , and observe no change in the noise level. Next, we consider whether the STM could describe the jitter in the resonator frequency. The central assumption of the STM is that certain atoms or groups of atoms may tunnel between two potential energy minima, which are separated in energy by an asymmetric splitting Δ 0 . The tunnelling coupling energy is given by Δ ~ e −λ , where λ is a tunnelling parameter proportional to the well separation and square root of the barrier height [2] . The Hamiltonian of each TLS has the form , where σ i ( i = x , y , z ) are the Pauli matrices. is the TLS energy splitting. The STM assumes that the energies Δ 0 and Δ are uncorrelated and have joint probability distribution: in a wide (atomic) range of energies, with typical density of TLSs, which is material-dependent. The TLSs interact with the external electric field and the strain field ε according to the Hamiltonian where is the electric dipole moment and γ is the elastic dipole moment. The effect of the interaction with the strain field can be seen as a renormalization of the asymmetry energy—that is, —therefore, it does not need to be treated separately. Different TLSs interact among themselves via long range dipole–dipole interaction (or phonon exchange) with an effective strength given by the dimensionless parameter with for electric (elastic) interactions. Here ? is the dielectric constant of the medium, ζ is the density of the glass and υ is the sound velocity. The dimensionless parameter is very small—that is, —such that within the STM interaction between TLS is assumed to be irrelevant. The dephasing and relaxation of the TLS is because of their interaction with phonons, giving a TLS relaxation rate , where k B is the Boltzmann constant. The probability distribution of due to the distribution of Δ and Δ 0 for a given E is wide and increases very rapidly near (ref. 26 ). Thermal fluctuations—absorption or emission of thermal phonons by an ensemble of independent TLSs—could cause a jitter in the resonator’s centre frequency (equivalent to a fluctuating dielectric constant Δ ε( r , t )). Since the number of activated TLSs is proportional to temperature and the effect of each TLS is small in T /ν 0 , the STM predicts [27] a noise spectrum that vanishes cubically for T << hν 0 /2 k B , in striking contrast to the results of Fig. 2 . Moreover, in the regime of strong applied electric field our calculations show that one should expect a very weak power dependence of the noise spectra, in disagreement with the results of Fig. 3b . As such, the STM is completely incompatible with our results. Other experimental studies have also found evidence for deviations from the STM. Individual TLS can be studied spectroscopically by superconducting qubits, allowing direct measurement of the relaxation time T 1 and the dephasing time T 2 of individual TLS [28] . The temperature dependence of these lifetimes has also been studied [20] , finding the expected wide distribution of relaxation rates for TLS, but in disagreement with STM predictions the temperature dependence of the relaxation rate is strong. Furthermore, the dephasing rate shows an anomalous behaviour: Γ 2 ~ T 1.24 . Studies of bulk ensembles of TLSs using high-Q superconducting resonators have also found deviations from STM predictions with resonators showing a logarithmic power dependence in contrast to the square root dependence predicted by the STM [29] , [30] . Second, the extracted density of states of TLS shows a weak power law dependence ρ ( E ) ∝ E μ , with μ =0.28 (manuscript in preparation). This is in agreement with several studies in glasses where a slight suppression of the density of states at low energies ρ ( E ) ∝ E μ with μ =0.3 was found [31] , [32] . Finally, it was found that in thin oxide a −SiO 2+ x layers, dipole–dipole interactions between TLSs may play a key role up to 100 mK [33] . All of this lead us to conclude that at least for thin oxide layers the STM does not correctly describe the properties of TLS. The generalized tunnelling model Our new model is conceptually shown in Fig. 1 : a resonator ( Fig. 1a ) with centre frequency ν 0 couples to an ensemble of coherent TLSs with energy-splitting hν 0 . Owing to non-negligible interactions with surrounding TLS, the resonant TLS acquire a temperature-dependent width and are affected by strongly coupled slow incoherent (classical) fluctuators ( Fig. 1b ). The latter causes an energy drift bringing the resonant TLS in and out of resonance. One key prediction of this new model is that it results in a low-frequency noise for a superconducting resonator that increases as the temperature is decreased. Moreover, this increase can be directly related to the microscopic parameter μ (introduced above), which is associated with the slight suppression of the density of TLS states at low energy. We argue that the noise observed in our measurements originates from thermally activated slow fluctuators that are also responsible for 1/ f charge noise in superconducting devices [34] . In particular, the resonator noise is generated by the switching of fluctuators that are located in the vicinity of quantum TLSs that are in resonance with the high-frequency electric field. In contrast to the STM, the interaction between TLSs is relevant for our model and the density of low-energy states is slightly non-uniform. In fact, any significant interaction between local degrees of freedom leads to the suppression of density of states at low energies. The effect is most dramatic for long-range Coulomb interaction in three dimensions where it leads to the E 2 dependence of the density of states known as the Efros–Shklovskii gap. Weaker but similar effect takes place for dipole–dipole interaction where similar arguments give a logarithmic energy suppression. It is not known whether higher orders of the perturbation theory give small power instead of the logarithm. It is also not excluded that experimental evidence for small power can be interpreted as a logarithmic correction. In this paper we adopt a phenomenological point of view that the density of states is described by a small-power law [35] , [36] . The assumption made in the STM that the size of the interaction is small is based on the hypothesis that the TLSs are local objects spaced at distances much larger than their size; however, this has never been proven experimentally—even for conventional glasses. (See Methods for details.) We now show qualitatively that the assumptions of the dominant role of TLS–TLS interaction and the energy-dependent density of states explain the present data as well as the results of phase qubit experiments [20] , [37] . Similarly to that of optical homogeneous linewidth [38] , the dephasing rate of the resonant TLS can be estimated by associating the dephasing process with the thermal relaxation of off-resonant TLSs that interact strongly with it. Since for a density of states ρ ( E ) ∝ E μ , the number of the off-resonant TLSs is proportional to T 1+ μ , the resulting width is Γ 2 ∝ T 1+ μ . Owing to this width, phononless relaxation processes between resonant TLSs become possible with rate Γ 1 ∝ T 1+ μ . Note that this power law is expected to hold at low temperature even while it dominates over the direct phonon emission. From our data we obtain μ ≈0.2–0.4; as a result we get an estimate for the dephasing rate in very good agreement with the value μ =0.24 obtained from measurements of phase qubits. Furthermore, the wide distribution of relaxation rates implies the presence of very slow TLSs in the vicinity of the resonant ones. These very slow TLSs have coherence times much shorter than the tunnelling rate and thus they can be considered as classical fluctuators. Their presence is independently revealed by charge fluctuations that display a 1/ f power spectrum [34] . The effect of the classical fluctuators on the resonant quantum TLSs is to generate an energy drift of the TLS with a 1/ f spectrum [29] . However, this only occurs if the interaction strength between the classical and coherent TLS is greater than the TLS width—that is, if the slow fluctuators are located within a distance R max =( U 0 / Γ 2 ) 1/3 from the resonant quantum TLS. An important consequence of this picture is that the noise increases as the temperature decreases. This is because of the fact that as the width decreases with temperature the energy drift becomes more visible. As a result, with decreasing temperature the noise sensitivity increases, even if the number of thermally excited fluctuators decreases. Analytical computations based on Bloch equations [39] give the following result for the noise spectrum: where N f is the number of strongly coupled fluctuators, is the Rabi frequency, is the applied electric field and V is the resonator volume. Using the measured value of μ ≈0.36 (see Fig. 2 ) allows this equation to describe all the results reported in this work. We emphasize the agreement of this value with that usually obtained for various glasses. Our model (see Methods) can also account for the power dependence (see Fig. 3b ). In fact, since Γ 1 Γ 2 ∝ T 2(1+ μ ) , the saturation term becomes temperature-dependent. For low powers, the spectra have an overall strong temperature dependence proportional to T −(1+ μ ) , whereas at high power our theory predicts that the temperature dependence of the spectra is constant. Figure 3b is a fit to the overall temperature and power dependence of the noise at 0.1 Hz: . In the fit, we used the measured value of μ ≈0.36; where A and B are sample-dependent parameters. We find that A ≈4 × 10 −16 for all temperatures. However, the value of B appears to change when the temperature is decreased below ~200 mK. For temperatures above 200 mK we find B =3.5 × 10 −3 and for temperatures below 200 mK we find B =2.5 × 10 −4 . As previously explained, the model is justified at lowest temperatures, so the observed cross-over between the two regimes is not surprising. Although saturation is seen at all temperatures in Fig. 3 , the saturation at the lowest temperature is the least clear. However, it should be noted that clear saturation in the low temperature limit has been observed elsewhere [18] . The results of this work can be instructive in identifying the nature of TLS. The remarkable agreement between the noise data and our model of strongly interacting TLS seems to indicate that in thin oxide layers the assumption of point-like defects needs to be revised. If TLSs are extended objects, the interactions between them can be significantly enhanced because they are effectively closer to each other and have a large dipole moment. The possibility of an extended nature of TLS was discussed, for example, in ref. 40 . In addition, the observed rise of 1/ f noise below ~1 K suggests that quantum devices, and in particular those comprising superconducting resonators, are not necessarily best operated at the lowest available temperatures. Instead, one should look for a sweet temperature spot with the largest signal-to-noise ratio or the longest coherence time. Finally, we note that the relevance of the interaction between TLSs in thin oxide layers does not contradict the existing body of data obtained previously on bulk amorphous materials. However, we do put forward the notion that results within literature on bulk materials may also benefit from a model including a dominant TLS–TLS interaction. Samples A 50-nm-thick epitaxial Nb film with a 5-nm Pt-capping layer was grown by laser ablation on r-plane sapphire substrate in an ultrahigh vacuum chamber with a base pressure of 10 −9 Torr and at a growth temperature of 650 °C. The typical Nb films grown under these conditions [41] were single-crystalline Nb (100) with low surface roughness, 0.3–0.5 nm. The film was patterned into an array of resonators coupled to a common feedline on a 10 × 5 mm 2 chip [17] , [30] using optical lithography and dry etching in a 2:1 ratio SF 6 /Ar plasma. The resonators used in our experiments are of the lumped element type, consisting of an inductive meander (inductance ~5 nH) in parallel with an interdigitated capacitor, see Fig. 1a . The centre frequency ( ν 0 ) of these resonators is in the 4- to 8-GHz band, and intrinsic quality factors ( Q i ) above 10 5 . Measurements A Pound frequency locked loop (described in detail in ref. 21 ) is used for all measurements. The high sensitivity and high bandwidth of this technique make it suitable for a variety of resonance measurements [42] , [43] including noise measurements [17] . The intrinsic loss tangent—proportional to the concentration and dipole moment of TLS—of the resonators tan Δ i was measured using the standard technique of fitting the ν 0 versus T dependence [30] . For both samples we find F tan Δ i , where F is a filling factor of order 1, to be around 1 × 10 −6 indicating very low dielectric loss. Additional epitaxial samples without the Pt-capping layer were found to exhibit similar parameters but with Q i ≲ 100,000 and F tan Δ I >2 × 10 −6 , which is similar to previous work using sputtered Nb [30] . The Pt-capping layer both increased Q i by a factor of 5 and significantly reduced the dielectric loss tangent. This improvement is probably because of the Pt minimizing the intrinsic oxide layer on the niobium surface. As predicted by the STM theory, the presence of TLS gives rise to temperature-dependent resonant frequency shifts. However, the low loss tangent in our samples meant that a ±10-mK-temperature fluctuation corresponds to a 200-Hz frequency shift, which is smaller than the flicker noise level at −100-dBm drive power [17] . Such insensitivity to temperature fluctuations is a stringent requirement for measuring the temperature dependence of any slow process, which could otherwise be masked by temperature-induced drifts. All measurements were performed in a well-shielded dilution refrigerator equipped with a cryogenic HEMT amplifier and heavily attenuated microwave lines. Our measurement setup has been described elsewhere, see refs 17 , 21 . Data analysis The measured data were processed by calculating the overlapping Allan deviation (ADEV) from the acquired time series. Each ADEV was then pre-screened for any signs of temperature drift, in which case the data set was discarded. By fitting to the 1/ f part of the ADEV, which for these sample occur for t >0.01 s, we then parametrize the frequency noise as S y ∝ h −1 / f , where S y is the fractional frequency spectra, and extract h −1 . This is then used to plot the data in the more familiar form as the noise level at 0.1 Hz (calculated from the h −1 value). Model The measured noise in the resonator is because of the coupling between the TLS electric dipole moment and the applied electric field of the resonator. Our model assumes that: (1) TLSs have the following probability distribution for the asymmetry energy Δ 0 and the tunnelling energy Δ : where and values of μ are discussed in the text. (2) TLS–TLS interactions are large and scale as 1/ r 3 (see below). These two assumptions are in contrast to the STM [1] , [2] where the asymmetry energy distribution is assumed to be constant and the interactions between TLSs are considered negligible. The large interaction between TLSs implies that a typical coherent TLS is strongly coupled to other coherent TLS. Here strongly coupled means that two TLSs have an interaction strength , where is the phonon-mediated relaxation rate for the TLS defined in the text. In this case, the mutual interaction results in an additional dephasing channel for the TLS. Calculations give a dephasing width Γ 2 ∝ T 1+ μ for TLS. In addition, strong interaction implies the presence of incoherent TLS (that is, classical fluctuators) strongly coupled to coherent TLS in resonance with the frequency of the resonator. Similarly to the coupling between coherent TLS, here strongly coupling means that U 0 r −3 > Γ 2 , so that slow fluctuators cause an energy drift for the resonant TLS: E ( t )= E +ξ( t ) with larger than the line width. Here N f denotes the number of strongly coupled flucutators, r k is the distance of the k -fluctuator to the resonant TLS and n k ( t )=±1 is a random telegraph signal with associated switching rate γ k . Note that these definitions of strong coupling imply that the scale of the interaction strength U 0 might be still very small in absolute terms. How to cite this article: Burnett, J. et al. Evidence for interacting two-level systems from the 1/ f noise of a superconducting resonator. Nat. Commun. 5:4119 doi: 10.1038/ncomms5119 (2014).